Pushing the limits of CMOS optical parametric amplifiers with USRN:Si7N3above the two-photon absorption edge CMOS platforms operating at the telecommunications wavelength either reside within the highly dissipative two-photon regime in silicon-based optical devices, or possess small nonlinearities. Bandgap engineering of non-stoichiometric silicon nitride using state-of-the-art fabrication techniques has led to our development of USRN (ultra-silicon-rich nitride) in the form of Si 7 N 3 , that possesses a high Kerr nonlinearity (2.8 × 10 −13 cm 2 W −1 ), an order of magnitude larger than that in stoichiometric silicon nitride. Here we experimentally demonstrate high-gain optical parametric amplification using USRN, which is compositionally tailored such that the 1,550 nm wavelength resides above the two-photon absorption edge, while still possessing large nonlinearities. Optical parametric gain of 42.5 dB, as well as cascaded four-wave mixing with gain down to the third idler is observed and attributed to the high photon efficiency achieved through operating above the two-photon absorption edge, representing one of the largest optical parametric gains to date on a CMOS platform. In the fields of attosecond nonlinear optics [1] , ultrafast laser spectroscopy [2] and precision manufacturing [3] , intense optical fields are required to approach the regimes of light necessary for the observation of both linear and nonlinear phenomena. When high powers are not directly available from electrically pumped lasers, amplification of light through rare-earth media [4] , [5] , semiconductor-based optical amplifiers [6] and Raman amplifiers [7] , [8] , [9] are adopted. Of the three aforementioned methods of amplification, rare-earth doped amplifiers are the most prolific at the telecommunications wavelength, where high gain may be achieved via down-conversion of light at the 980 to the 1,550 nm region. In the context of complementary metal–oxide–semiconductor (CMOS)-based photonics systems, rare-earth doped amplifiers have not proliferated to the extent that they have in fibre-based technologies, possibly due to the difficulty in doping CMOS materials with erbium while maintaining sufficiently low losses. Raman amplifiers, which leverage phonon–photon interactions to amplify light at a wavelength, which is up- or down-shifted from a wavelength corresponding to the Raman shift in the medium, have seen considerable success in waveguide platforms, particularly in silicon-based Raman amplifiers [8] , [9] . However, the narrowband Raman gain spectrum within crystalline materials such as silicon precludes the amplification of optical fields possessing wide spectral bandwidths such as ultrafast pulses. In addition, since the gain in Raman-based amplifiers obeys a power law with respect to the pump power, significant pump powers are required for high gain. Similar to Raman amplifiers, optical parametric amplifiers also rely on the inherent nonlinearity of the host medium to achieve optical amplification. While Raman amplifiers rely on a large Raman coefficient for gain, optical parametric amplifiers utilize the Kerr nonlinearity inherent in the host medium [10] . Contrary to rare-earth doped and Raman amplifiers, where the gain wavelength is fixed with respect to the pump wavelength, optical parametric amplification allows for an additional design degree of freedom, where light at carefully designed wavelengths may be engineered to undergo amplification via the transfer of photons from the pump. In this process, conservation of momentum is satisfied via phase matching techniques, which have advanced significantly to now cover approaches such as tailoring of waveguide geometries [11] , [12] , [13] , [14] , [15] , [16] , quasi-phase-matched structures [17] , [18] , metamaterials [19] and first-principles materials synthesis [20] . In addition to the ability for optical parametric amplifiers to amplify light at a large range of wavelengths with respect to the pump, the amplified signals scale quadratically with the pump power, enabling extremely large amplification factors. Optical parametric amplification with high gain is therefore highly sought after, as it is one of the most efficient methods for amplifying light and achieving high-powered optical fields; apart from the aforementioned applications in attosecond nonlinear optics, ultrafast laser spectroscopy and precision manufacturing, within the burgeoning field of CMOS photonics, devices capable of high conversion efficiencies or parametric amplification are likely to find their place as compact, multi-wavelength sources necessary to significantly reduce the high per unit costs of lasers used to power wavelength division multiplexing-based transceivers, or provide compensatory amplification. Fundamental to optical parametric amplification within centrosymmetric materials is its inherent Kerr nonlinearity. Large optical nonlinearities and negligible nonlinear losses are ideal for such processes, as they enable the parametric process to occur efficiently using low power [21] . In addition to the Kerr nonlinearity of the material, absorptive mechanisms that compete with the amplification process need to be kept to a minimum. The body of work surrounding CMOS nonlinear optics suggests strongly that operating outside of the two-photon absorption regime is necessary to maintain high photon efficiencies. While two-photon processes are desirable for a variety of applications such as microscopy [22] , [23] , pulse characterization [24] and nanofabrication [25] , this absorptive mechanism needs to be mitigated in Kerr-based nonlinear processes. The three-photon absorption cross-section is typically much smaller than the two-photon absorption cross-section [26] . Consequently, nonlinear losses can be well reduced by operating in the three-photon rather than two-photon regime. To date, demonstrations of CMOS-based optical parametric amplifiers at the telecommunications wavelength have been limited to platforms possessing non-negligible two-photon and free-carrier losses [27] , [28] , [29] . Consequently, maintaining a high photon efficiency while simultaneously possessing the large parametric gain required for most practical applications such as integrated light sources for transceivers or active optical cables continues to be an important element in CMOS-based optoelectronics. Having identified the limitations in existing CMOS platforms, and the requirements for achieving high parametric gain with high photon efficiencies, we recently developed a proprietary nonlinear material especially for this purpose, where guided by design rules from Kramers–Kronig relations [30] and Miller’s rule [31] , we have succeeded in creating ultra-silicon-rich nitride (USRN), which has a material composition of Si 7 N 3 (more details in Supplementary Note 1 ), possessing one of the largest optical nonlinearities of any CMOS material to date, in which two-photon absorption is still absent—ideal qualities for realizing high gain optical parametric amplifiers. In this paper, we demonstrate 42.5 dB optical parametric gain using a CMOS waveguide designed to achieve phase matching across a broad bandwidth. This gain represents one of the highest gains at the telecommunications wavelength to date. High photon efficiencies are demonstrated as a result of the platform composition, tailored to have a wide enough bandgap to eliminate two-photon absorption, including that from Urbach tails, while maintaining a large linear and nonlinear refractive index to achieve optimum gain. High gain is achieved owing to the large Kerr nonlinearity, high field localization within the designed device and negligible nonlinear losses. Design rules for the highly nonlinear Si 7 N 3 platform Kramers–Kronig relations describe the causal relationship between the real and imaginary parts of a material’s dielectric constant [30] . Two important insights offered by the Kramers–Kronig relations is the peaking of a material’s refractive index close to its bandgap wavelength, and the reduction in nonlinear absorption as the bandgap is increased. Photon–electron dynamics are strongly dependent on a material’s bandgap, and offer further insight into the derivative refractive index. Photons incident on a medium at a frequency larger than its bandgap are optically absorbed, and cause electrons to cross into the conduction band. Materials with larger bandgaps, namely insulators, have electrons that are tightly bound to the atom, and any incident photon below the bandgap energy does not interact strongly with the electrons. This implies that the impact of photon–electron interactions on the medium’s refractive index is minimal. As the bandgap decreases to that, say, of a semiconductor, electrons are now less tightly bound to the atom and experience moderate interaction with an incident photon. This interaction effectively retards the movement of the photon through the medium thus leading to a larger refractive index. Consequently, interactions between incident photons and electrons within the material govern the inverse relationship between material bandgap and linear refractive index. Similar to the impact of photon–electron interactions on the linear refractive index, the nonlinear polarizability of a material also increases with a decreasing bandgap, a phenomenon that is also empirically described by Miller’s rule [31] . Therefore, it appears that there is an optimum material property with a tailored composition between silicon nitride and amorphous silicon, where the bandgap is sufficiently large to position the 1,550 nm wavelength in the significantly less dissipative multi-photon regime without two-photon absorption effects from Urbach tails, while maintaining a large nonlinearity. CMOS-based platforms in particular are especially important for their large-scale manufacturability and ease of integration with CMOS electronics. A continuum of silicon-based CMOS materials from silicon dioxide ( n ∼ 1.46) to amorphous silicon ( n as high as 4.0) are actively being studied as nonlinear optical platforms, each possessing different pros and cons. In amorphous silicon devices where bandgaps as large as 1.7 eV have been demonstrated for nonlinear optics devices, two-photon absorption has been reported to exist from residual Urbach tails [32] , [33] , [34] . Increasing the bandgap further could similarly yield nonlinear devices with better nonlinear figures of merit [35] . In Fig. 1 , we summarize a few CMOS-based amorphous oxide- and nitride-based silicon materials plotted with refractive index and bandgap against the nonlinear refractive index, which follows a log-linear scaling rule. Consistent with Kramers–Kronig and Miller’s rule, as we move up the refractive index scale, bandgap energy decreases and the nonlinear refractive index increases. Guided by these design rules, our current endeavour establishes a new paradigm in nonlinear CMOS optics research, where we have succeeded in synthesizing USRN:Si 7 N 3 . The term USRN is adopted to distinguish this material from other silicon-rich nitride films, which are characterized by a lower linear (typically ≤2.2 versus 3.1 in USRN) and nonlinear refractive index, and considerably less silicon-rich than our films [36] , [37] , [38] , [39] , [40] . Our USRN films possesses one of the largest optical nonlinearities of any CMOS material to date, and in which two-photon absorption is still absent, ideal qualities for realizing high-gain optical parametric amplifiers. 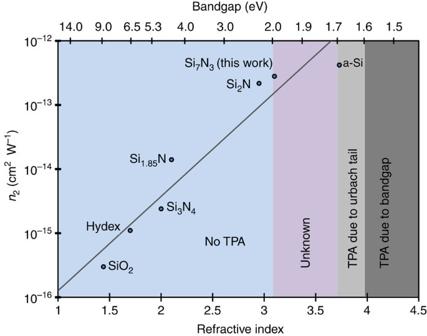Figure 1: List of CMOS amorphous solids on a refractive index scale. Values are taken from refs13,20,28,29,33,34,35,36,37,38,39,40,43,50,53,55,65,66. The nonlinear refractive index and bandgap energies for each material follow a scaling rule as indicated by the grey solid line as a guide to the eye. The bandgap relation to the refractive index is fitted empirically with reported values. Materials in grey reside in the two-photon absorption (TPA) regime at 1,550 nm. Figure 1: List of CMOS amorphous solids on a refractive index scale. Values are taken from refs 13 , 20 , 28 , 29 , 33 , 34 , 35 , 36 , 37 , 38 , 39 , 40 , 43 , 50 , 53 , 55 , 65 , 66 . The nonlinear refractive index and bandgap energies for each material follow a scaling rule as indicated by the grey solid line as a guide to the eye. The bandgap relation to the refractive index is fitted empirically with reported values. Materials in grey reside in the two-photon absorption (TPA) regime at 1,550 nm. Full size image Continuous-wave four-wave-mixing experiments To characterize the ability of the designed USRN waveguides to perform parametric wavelength conversion, four-wave-mixing experiments are first performed using a continuous-wave pump and signal as a precursor to the demonstration of optical parametric amplification. 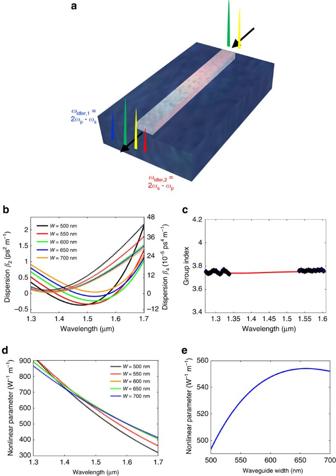Figure 2: Device schematic and optical properties of the USRN waveguides. (a) Schematic of the ultra-silicon-rich nitride waveguides used to perform four-wave-mixing experiments. (b) The calculated second-order (β2, solid lines) and fourth-order (β4, dashed lines) dispersion of the USRN waveguides for different waveguide widths (W). The USRN waveguide height is fixed at 300 nm. (c) Measured and calculated group index of the fabricated USRN waveguide. (d) Calculations of the nonlinear parameter of the waveguide as a function of wavelength for various waveguide widths (W) and fixed waveguide height of 300 nm. (e) Nonlinear parameter as a function of waveguide width for a pump at 1,550 nm. The values of the measuredn,kvalues of the USRN films are used in the dispersion and nonlinear parameter calculations. Figure 2a shows a pump and signal entering the USRN waveguide, and generating phase-matched idlers through the four-wave-mixing process. USRN waveguides, 550 nm wide and 300 nm high with a length of 7 mm, are first fabricated using 300 nm-thick USRN films (see Methods and Supplementary Note 1 ). Figure 2b shows the calculated dispersion for the quasi-transverse electric mode. The waveguides’ second-order dispersion ( β 2 ) and fourth-order dispersion ( β 4 ), may be calculated using [21] and respectively, where , ω is the angular frequency, c is the speed of light in vacuum and n g is the group index of the waveguide. To measure the dispersion of the waveguide, the group index of the waveguide is extracted using a method similar to that used in ref. 13 . Within the 1,520–1,610 nm wavelength range, fringe visibility is excellent and this enables us to easily observe that the group index increases gradually, implying anomalous dispersion. For comparison, the extracted group index data for the wavelength range between 1,250 and 1,310 nm is also shown in Fig. 2c , where the group index also matches well with the calculated value. The fringe visibility in this case however is not as good as that within the 1,520–1,610 nm wavelength range. The extracted average waveguide dispersion between 1,520 and 1,610 nm is characterized to be 0.28 ps 2 m −1 or 200 ps nm −1 km −1 , which is very close to the calculated value of 120 ps nm −1 km −1 within this wavelength region ( Fig. 2c ). For completeness, numerical calculations of the nonlinear parameter of the waveguides are performed using the expression Figure 2: Device schematic and optical properties of the USRN waveguides. ( a ) Schematic of the ultra-silicon-rich nitride waveguides used to perform four-wave-mixing experiments. ( b ) The calculated second-order ( β 2 , solid lines) and fourth-order ( β 4 , dashed lines) dispersion of the USRN waveguides for different waveguide widths ( W ). The USRN waveguide height is fixed at 300 nm. ( c ) Measured and calculated group index of the fabricated USRN waveguide. ( d ) Calculations of the nonlinear parameter of the waveguide as a function of wavelength for various waveguide widths (W) and fixed waveguide height of 300 nm. ( e ) Nonlinear parameter as a function of waveguide width for a pump at 1,550 nm. The values of the measured n , k values of the USRN films are used in the dispersion and nonlinear parameter calculations. Full size image where k 0 is the free-space wave vector and n 2 (previously measured to be 2.8 × 10 −13 cm 2 W −1 in ref. 41 ) is the nonlinear refractive index of the USRN film, are also included in Fig. 2d,e . Four-wave-mixing experiments are first performed using a low continuous-wave pump power of 4.7 dBm centred at 1,555 nm and a continuous-wave signal, while the signal wavelength is varied. 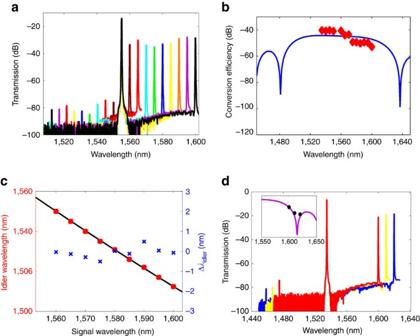Figure 3: Broadband low power parametric wavelength conversion in USRN waveguides. (a) Generated four-wave-mixing spectra as the signal wavelength is tuned from 1,560 to 1,610 nm using a pump located at 1,555 nm. Solid lines denote the four-wave-mixing spectra for a signal located at 1,560 (brown), 1,565 (red), 1,570 (cyan), 1,575 (green), 1,580 (blue), 1,585 (yellow), 1,590 (orange), 1,595 (purple) and 1,600 nm (black). (b) Calculated (blue solid line) and measured (red squares) conversion efficiency as a function of signal wavelength, using a pump located at 1,555 nm. (c) Measured (red squares) and calculated (black solid line) idler wavelength as a function of the signal wavelength. (d) Four-wave mixing using a pump at 1,535 nm and signal at 1,620 nm representing conversion over 170 nm. Solid lines denote the four-wave-mixing spectra for a signal located at 1,600 (red), 1,610 (yellow) and 1,620 nm (blue). Inset shows the calculated (purple line) and measured (black diamonds) conversion efficiency as a function of wavelength. Figure 3a shows plots of the generated idler. A peak conversion efficiency of −40 dB is achieved using this pump power. The wavelength of the signal was tuned and conversion to the anti-Stokes side was observed for signal wavelengths from 1,535 to 1,610 nm. Conversion over 90 nm is observed using this pump wavelength. Figure 3: Broadband low power parametric wavelength conversion in USRN waveguides. ( a ) Generated four-wave-mixing spectra as the signal wavelength is tuned from 1,560 to 1,610 nm using a pump located at 1,555 nm. Solid lines denote the four-wave-mixing spectra for a signal located at 1,560 (brown), 1,565 (red), 1,570 (cyan), 1,575 (green), 1,580 (blue), 1,585 (yellow), 1,590 (orange), 1,595 (purple) and 1,600 nm (black). ( b ) Calculated (blue solid line) and measured (red squares) conversion efficiency as a function of signal wavelength, using a pump located at 1,555 nm. ( c ) Measured (red squares) and calculated (black solid line) idler wavelength as a function of the signal wavelength. ( d ) Four-wave mixing using a pump at 1,535 nm and signal at 1,620 nm representing conversion over 170 nm. Solid lines denote the four-wave-mixing spectra for a signal located at 1,600 (red), 1,610 (yellow) and 1,620 nm (blue). Inset shows the calculated (purple line) and measured (black diamonds) conversion efficiency as a function of wavelength. Full size image The conversion efficiency taking into account the waveguide nonlinear parameter, second- and fourth-order dispersion and propagation losses is calculated as a function of wavelength for a pump at 1,555 nm and signal at 1,560 nm, and shown in Fig. 3b , together with the measured conversion efficiency. By energy and momentum conservation, the wavelength of the generated idler is governed by the expression, ω idler =2 ω pump − ω signal (ref. 21 ). Figure 3c plots the calculated and measured idler wavelengths, as well as the deviation from the calculated idler wavelength. It is observed that there is a good match between the calculated and measured idler wavelengths. The deviation between the calculated and measured idler wavelengths is <0.5 nm for all measured signal wavelengths, which is further evidence that energy transfer from the pump and signal to the idler on the anti-Stokes side is occurring through the four-wave-mixing process. To further investigate the achievable conversion bandwidth, we use a pump wavelength of 1,535 nm, and increase the signal wavelength. The generated idler is shown in Fig. 3d . Importantly, we were able to observe parametric conversion for signal wavelengths as high as 1,620 nm. This represents a broadband wavelength conversion over 170 nm. Next, four-wave mixing using a pump at 1,560 nm and a signal at 1,555 nm was performed. The conversion efficiency as a function of the pump power was tracked by monitoring the idler power at 1,565 nm. 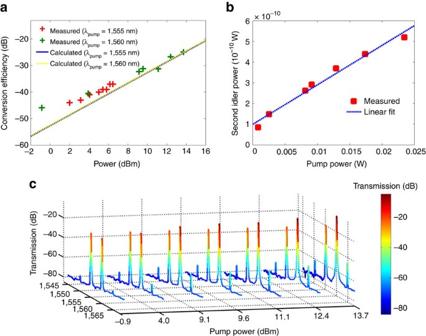Figure 4: Characterization of the USRN waveguide conversion efficiency. (a) Measured conversion efficiency as a function of pump power. Blue solid and yellow dashed lines represent the calculated conversion efficiency as a function of pump power for a pump wavelength of 1,555 and 1,560 nm, respectively. (b) Four-wave-mixing experiments using a pump at 1,560 nm and a signal at 1,555 nm. (c) Evolution of the spectrum measured at the USRN waveguide output as the pump power (at 1,560 nm) is increased. The first and second idler powers are observed to increase with pump power. Figure 4a shows the conversion efficiency as a function of the pump power, together with the theoretically expected conversion efficiency. The maximum conversion efficiency obtained with the power levels used in this experiment was −24.9 dB, corresponding to a pump power of 13.7 dBm. It is observed that the conversion efficiency increases as the pump power is increased along the same trajectory as that which is theoretically expected. This result further implies that nonlinear losses at the wavelengths and power levels used in the experiment are negligible, and the expected dominant multi-photon nonlinear loss mechanism (three-photon absorption) is not observed. Figure 4: Characterization of the USRN waveguide conversion efficiency. ( a ) Measured conversion efficiency as a function of pump power. Blue solid and yellow dashed lines represent the calculated conversion efficiency as a function of pump power for a pump wavelength of 1,555 and 1,560 nm, respectively. ( b ) Four-wave-mixing experiments using a pump at 1,560 nm and a signal at 1,555 nm. ( c ) Evolution of the spectrum measured at the USRN waveguide output as the pump power (at 1,560 nm) is increased. The first and second idler powers are observed to increase with pump power. Full size image Parametric wavelength conversion for the idler on the Stokes side, which we refer to here as the second idler, is described by the phase-matching condition, ω idler, Stokes =2 ω signal − ω pump . Similar to conversion to the first idler, this process is also degenerate, but at the signal wavelength instead of the pump wavelength. In this case, two photons at the signal wavelength are annihilated to yield one photon at the pump wavelength and one at the idler on the Stokes side. As a result of this conversion process being degenerate at the signal wavelength, the power at the second idler follows a linear dependence with the input pump power, and a quadratic dependence with the signal power. Figure 4b shows the measured power at the second idler, generated at a wavelength of 1,550 nm, as a function of the pump power. The measured idler power closely follows a linear relationship with the pump power, in agreement with the expected behaviour of the parametric conversion process. The evolution of the generated first and second idler is also shown in Fig. 4c , showing the increase in idler power as the pump power is increased. High-gain optical parametric amplification is best achieved in media with a high nonlinear parameter and negligible losses. Through the four-wave-mixing experiments, large conversion efficiencies are achieved across a broad bandwidth at modest power levels. No saturation in the conversion efficiency is observed at the power levels used, implying that nonlinear losses are negligible. Previous experiments using short pulses also verified that nonlinear losses at the 1.55 μm wavelength are negligible in our USRN waveguides for intensities up to 50 GW cm −2 (ref. 41 ). Optical parametric amplification experiments Previous demonstrations of optical parametric amplification in CMOS platforms at the telecommunications wavelength are limited mainly to platforms possessing non-negligible two-photon and free-carrier effects. The first demonstration of optical parametric amplification in crystalline silicon was performed at the telecommunications wavelength, where two-photon and free-carrier losses are still present, and limited the on/off parametric gain to 5 dB (ref. 27 ). Following this work was a demonstration of optical parametric amplification in crystalline silicon at the two-photon absorption edge of 2,200 nm (ref. 42 ). Close to this wavelength, the two-photon coefficients become negligible and the three-photon absorption coefficient ∼ 3 × 10 −22 cm 3 W −2 (ref. 26 ), and becomes the dominant nonlinear absorption mechanism. Consequently, on/off parametric gain of close to 30 dB was achieved at the mid-infrared with 33 W of peak pump power. More recently, amorphous silicon has been used as a platform for 26.5 dB of on/off parametric gain, though through the use of a pulsed signal and pump to overcome spatio-temporal build-up of photo-excited free-carriers [28] . On/off parametric gain of 11 dB using a continuous-wave signal has recently been achieved. However, sub-nanosecond carrier lifetimes in amorphous silicon have also been shown to saturate four-wave-mixing conversion efficiencies at powers larger than 15 mW (refs 29 , 43 ). Clearly, the presence of two-photon and free-carrier absorption in any platform will limit the optical parametric amplification process. As an illustration of the importance of low nonlinear losses, chalcogenide waveguides with low nonlinear losses [44] , [45] , [46] , although not CMOS compatible, have also been used at the telecommunications wavelength to demonstrate a large net off-chip gain of 16 dB (ref. 45 ). Optical parametric amplification experiments are performed using our USRN device using a pulsed pump and a continuous-wave signal. The mixing of two pump photons and one signal photon generates one idler photon. Since the pump is pulsed, the mixing process occurs at a rate equivalent to the repetition rate of the laser, and the generated idler and amplified signal also assume a pulsed nature with the same repetition rate. In the first set of experiments, 500 fs pulses centred at 1,560 nm with a peak power of 14 W are combined with a continuous-wave signal (power fixed at 40 μW) using a wavelength division multiplexer. The signal wavelengths are varied from 1,620 to 1,630 nm, and the generated four-wave-mixing spectra is shown in Fig. 5a . Analyses of the on/off optical parametric gain experienced by the signal and idlers are performed ( Fig. 5b ) and details of parametric gain calculations are provided in Methods. The maximum parametric gain experienced by the signal and first idler is 42.5 and 36.2 dB, respectively. This signal gain, to our knowledge, represents the largest demonstrated to date on a CMOS compatible platform. 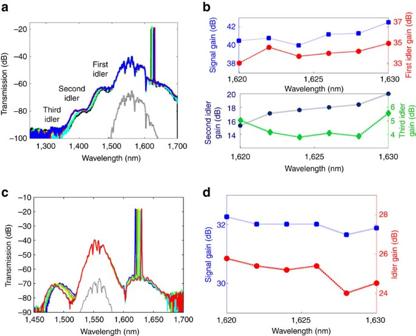Figure 5: Optical parametric-amplification and cascaded four-wave mixing using a 500 fs pump. (a) Transmission spectrum as a function of wavelength for a peak pump power of 14 W. Cascaded four-wave mixing down to the third idler at 1,300 nm is observed. Solid lines denote the measured spectra with the signal located at 1,620 (black), 1,622 (green), 1,624 (cyan), 1,626 (yellow), 1,628 (blue) and 1,630 nm (red). The grey dashed curve represents the pump spectrum offset by −25 dB, with the signal off. (b) Measured parametric gain in the signal (blue squares), first (red circles), second (dark blue stars) and third idlers (green diamonds). (c) Transmission spectrum as a function of wavelength for a peak pump power of 10 W. Solid lines denote the measured spectra with the signal located at 1620 (blue), 1,622 (orange), 1,624 (green), 1,626 (yellow), 1,628 (cyan) and 1,630 nm (red). The grey dashed curve represents the pump spectrum offset by −25 dB, with the signal off. (d) Measured signal (blue squares) and idler gain (red circles) as a function of signal wavelength. Dotted lines inb,dare a guide to the eye. Figure 5: Optical parametric-amplification and cascaded four-wave mixing using a 500 fs pump. ( a ) Transmission spectrum as a function of wavelength for a peak pump power of 14 W. Cascaded four-wave mixing down to the third idler at 1,300 nm is observed. Solid lines denote the measured spectra with the signal located at 1,620 (black), 1,622 (green), 1,624 (cyan), 1,626 (yellow), 1,628 (blue) and 1,630 nm (red). The grey dashed curve represents the pump spectrum offset by −25 dB, with the signal off. ( b ) Measured parametric gain in the signal (blue squares), first (red circles), second (dark blue stars) and third idlers (green diamonds). ( c ) Transmission spectrum as a function of wavelength for a peak pump power of 10 W. Solid lines denote the measured spectra with the signal located at 1620 (blue), 1,622 (orange), 1,624 (green), 1,626 (yellow), 1,628 (cyan) and 1,630 nm (red). The grey dashed curve represents the pump spectrum offset by −25 dB, with the signal off. ( d ) Measured signal (blue squares) and idler gain (red circles) as a function of signal wavelength. Dotted lines in b , d are a guide to the eye. Full size image One of the features within the measured spectrum, which shows the high nonlinearity and low nonlinear losses of the waveguide, is the evidence of cascaded four-wave mixing. This effect has also been observed in silicon at mid-infrared wavelengths, but not at the telecommunications wavelength. In this set of experiments, the third idler generated at the anti-Stokes side of the pump extends the spectrum all the way to 1,300 nm. The amplified signal peak power exceeds 100 mW, and enables efficient mixing with photons from other components generated through the four-wave-mixing process. Each generated idler serves as a possible source of photons from which to mix with photons at another wavelength and in so forth, undergo parametric conversion. The peak parametric gain extracted for the second idler is 21.2 dB, whereas that for the third idler is extracted to be 7.7 dB. Reducing the peak pump power to 10 W yielded a second set of four-wave-mixing spectra shown in Fig. 5c with each of the amplified signals and idlers possessing lower power. The maximum signal and idler gain in this case was measured to be 32.3 and 25.8 dB, respectively ( Fig. 5d ). In platforms possessing two-photon and free-carrier absorption, using pulses with short temporal widths has been shown to reduce (but not eliminate) their impact on nonlinear optical processes [47] , [48] , [49] , [50] . Experiments with continuous-wave light experience the greatest compromise in performance, due to a large free-carrier build-up [50] , [51] . Shorter pulses at smaller repetition rates allow free carriers to somewhat dissipate before the next pulse arrives. Within a single pulse, free carriers generated by the leading edge of the pulse tend to attenuate the trailing edge and also impart a nonlinear phase from the free-carrier dispersive effect. Consequently, pulses that are longer experience two-photon- and free-carrier-induced degradation in nonlinear performance to a greater extent [47] , [48] , [49] , [50] . We further investigate the ability of our designed devices to parametrically amplify light using longer pulses, to study the impact, if any, of nonlinear losses. Using pulses with a temporal duration of 2.0 ps centred at 1,560 nm, and a peak pump power of 10 W, four-wave-mixing experiments are performed and shown in Fig. 6 . In the regime of negligible nonlinear losses, the parametric gain should remain unchanged when the pulse width is varied (from 500 fs to 2.0 ps), but peak power is maintained. 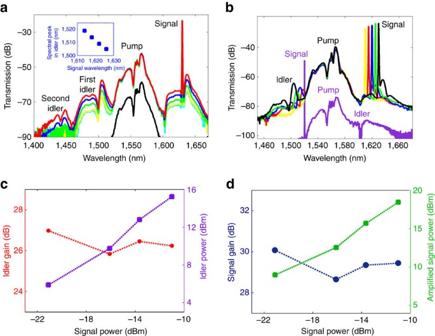Figure 6: Optical parametric amplification and cascaded four-wave mixing using a 2.0 ps pump. (a) Transmission spectrum as a function of signal power. The power of the generated idler scales linearly with the signal power. The spectral feature at 1,400–1,450 nm represents evidence of cascaded four-wave mixing. The black solid curve represents the pump spectrum offset by −15 dB, without the signal turned on. Coloured lines represent the measured spectra with a signal power of −21.1 (cyan), −16.1 (yellow), −13.7 (green) and −11.0 dBm (blue). The inset shows the location of the spectral peak in the first idler as a function of signal wavelength. (b) Measured four-wave-mixing spectra as the signal wavelength is tuned from 1610 to 1,630 nm, and 1,520 nm. Solid lines denote the measured spectra for a signal located at 1,610 (yellow), 1,615 (red), 1,620 (blue), 1,625 (green) and 1,630 nm (black). The spectrum for a signal at 1,520 nm is offset by −30 dB for clarity. (c) Measured idler gain (red circles) and power (purple squares) as a function of signal power at the waveguide output when the pump is off. (d) Measured amplified signal gain (blue circles) and power (green squares) as a function of signal power at the waveguide output when the pump is off. Dotted lines inc,dare a guide to the eye. Figure 6a shows the measured four-wave-mixing spectra including the observation of cascaded four-wave mixing up to the second idler. A peak parametric gain of 30 dB is achieved for the amplified signal. The gain for both the idler and signal is observed in Fig. 6c,d to remain relatively constant as the signal power is increased. The absence of any observable build-up of photo-excited free carriers and 30 dB parametric gain in the mixing of the pulsed-pump and continuous-wave signal implies that the demonstrated nonlinear effects are intrinsically ultrafast. Comparing the two experiments with the same peak power of 10 W but with different pulse durations (2.0 ps and 500 fs), a similar parametric gain is observed. This result is consistent with that expected from the negligible nonlinear losses experienced by the device at these power levels. For completeness, the four-wave-mixing spectra as the signal wavelength is varied from 1,610 to 1,630 nm is shown in Fig. 6b . Figure 6: Optical parametric amplification and cascaded four-wave mixing using a 2.0 ps pump. ( a ) Transmission spectrum as a function of signal power. The power of the generated idler scales linearly with the signal power. The spectral feature at 1,400–1,450 nm represents evidence of cascaded four-wave mixing. The black solid curve represents the pump spectrum offset by −15 dB, without the signal turned on. Coloured lines represent the measured spectra with a signal power of −21.1 (cyan), −16.1 (yellow), −13.7 (green) and −11.0 dBm (blue). The inset shows the location of the spectral peak in the first idler as a function of signal wavelength. ( b ) Measured four-wave-mixing spectra as the signal wavelength is tuned from 1610 to 1,630 nm, and 1,520 nm. Solid lines denote the measured spectra for a signal located at 1,610 (yellow), 1,615 (red), 1,620 (blue), 1,625 (green) and 1,630 nm (black). The spectrum for a signal at 1,520 nm is offset by −30 dB for clarity. ( c ) Measured idler gain (red circles) and power (purple squares) as a function of signal power at the waveguide output when the pump is off. ( d ) Measured amplified signal gain (blue circles) and power (green squares) as a function of signal power at the waveguide output when the pump is off. Dotted lines in c , d are a guide to the eye. Full size image Over the last few years, CMOS platforms with ultra-low linear losses and negligible nonlinear losses at 1.55 μm such as Hydex glass and silicon nitride have made great progress in nonlinear optics applications. Within the scope of nonlinear waveguide devices, the figure of merit, γ × L eff, max , where L eff, max =1/ α is the maximum effective length achievable in a waveguide with a loss coefficient of α , and γ is the nonlinear parameter, provides a metric for comparison between nonlinear waveguides, where the acquired nonlinear phase scales linearly with the incident peak power (negligible nonlinear losses). The figures of merit γ × L eff, max for Hydex glass [52] (loss=0.06 dB cm −1 and γ ∼ 0.22 W −1 m −1 ), and ultra-low-loss silicon nitride in ref. 53 (loss=0.06 dB cm −1 and γ ∼ 0.29 W −1 m −1 ) and ref. 54 (loss=0.5 dB cm −1 and γ ∼ 1 W −1 m −1 ) are calculated to be 0.16, 0.21 and 0.087 W −1 , respectively. For the USRN waveguides used in this work to achieve 42.5 dB of optical parametric gain (loss=4.5 dB cm −1 and γ ∼ 500 W −1 m −1 ), γ × L eff, max =4.8 W −1 , which suggests that nonlinear waveguide devices implemented on this platform, are able to achieve close to 30 times more nonlinear phase than ultra-low-loss platforms at the same peak power level. The performance comparison becomes more complicated when considering the use of resonator enhancement. Because resonators typically possess a very narrow resonance bandwidth, they are best suited to applications that do not require the manipulation of broadband signals, such as low-power nonlinear switching of continuous-wave signals or optical frequency combs. Resonators with high-quality factors increase the effective optical path length while maintaining a small device footprint, generate a power enhancement within the resonator, and offer the greatest advantages when utilized on platforms with negligible nonlinear losses such as Hydex glass and silicon nitride. Silicon-based resonators, for example, have been limited to conversion efficiencies of −39 dB (ref. 51 ) as a result of nonlinear losses, and this has precluded the realization of on-chip silicon-based optical parametric oscillators at 1.55 μm. Hydex glass and silicon nitride have shown excellent performance: experimental reports of continuous-wave four-wave mixing in Hydex waveguides, using high- Q resonators, utilized 5 mW of pump power to realize −46 dB of conversion efficiency [55] . Resonators with large quality factors of 1.2 × 10 6 and 5 × 10 5 , with pump powers of 101 (ref. 52 ) and 50 mW (ref. 54 ), respectively, have further been used to achieve optical parametric oscillation. Because of the twofold effect of resonator power enhancement and augmented effective optical path length, nonlinear phase from a resonator scales with the square of the finesse, F ( versus ) (ref. 56 ). An estimation of F 2 for the devices used in refs 52 , 54 show that Hydex glass and silicon nitride possess a large F 2 ∼ 10 6 , enabling resonator enhancements to the nonlinear phase acquisition by this factor. As a result of their ultra-low losses, both Hydex glass and silicon nitride resonators offer significant enhancements in nonlinear phase acquisition, two orders of magnitude greater than that in our USRN platform ( F 2 ∼ 10 4 ) [41] , and have been successfully configured as nonlinear resonator-enhanced devices for high-performance frequency combs [57] , [58] , [59] , [60] , [61] , [62] . Further reductions in propagation losses could enable resonators on the USRN platform to approach these levels of resonator enhancement. It was previously postulated that material losses in nitride-based CMOS materials deposited at low temperatures possessed high material losses at 1.55 μm because of absorption from N–H and Si–H bonds at that wavelength [13] , [57] . To further evaluate the material losses of our USRN films, ellipsometric measurements with an accuracy of 10 −6 in the measured k value were performed ( Supplementary Fig. 1f ). The k value measured at the 1.55 μm region is below the minimum measurable k value, which implies that the USRN material loss is lower than 0.35 dB cm −1 . Similar to other high confinement waveguides such as silicon on insulator waveguides, fabrication-induced sidewall scattering plays a role in waveguide losses. Experiments to quantify the losses of the waveguides reveal an inverse relationship between the linear waveguide loss and the waveguide width. In waveguides where the width was increased to 700 nm, losses as low as 1.9 dB cm −1 were measured ( Supplementary Fig. 1e ), which suggest that further optimizations in fabrication processes could yield even lower losses, to approach the levels of resonator enhancement available in ultra-low loss platforms. We have experimentally demonstrated 42.5 dB optical parametric gain at the telecommunications wavelength using USRN. This represents the largest optical parametric gain at this wavelength to date on a CMOS platform. In addition, cascaded four-wave mixing with gain is observed up to the third idler, and low power, continuous-wave four-wave mixing on the USRN waveguides are also demonstrated. Broadband conversion from 1,620 to 1,460 nm is facilitated by the ability to achieve substantial conversion efficiencies using short waveguides while keeping within the coherence length, with peak conversion efficiencies of −24.9 dB using 13.7 dBm of pump power. By engineering the films to reside outside the two-photon regime and well within the multi-photon regime, the USRN waveguides possess the ideal combination of a large nonlinearity and nonlinear losses below the detection limit at the 1,550 nm wavelength, while being compatible with back-end CMOS processing. Future developments on this platform could yield applications in high-performance nonlinear optical pulse compressors and low power, ultra-broadband light sources. USRN growth We engineer the USRN films using inductively coupled plasma chemical vapour deposition. USRN films are deposited at a low temperature of 250 °C, making them suitable for back-end CMOS processing. USRN films of up to 2 μm in thickness have been successfully deposited without noticeable cracks or stress-related bending. Detailed studies into the film growth are provided in ref. 20 . Precursor gases used are SiH 4 and N 2 ; NH 3 is intentionally avoided as it is likely to generate unwanted N–H bonds, which have absorption peaks close to the 1.55 μm wavelength [63] . Material studies of the films were performed using X-ray photo-electron spectroscopy to determine the film composition, presence of silicon and nitrogen in the films and information pertaining to the energy bandgap. Further details are available in Supplementary Note 1 . USRN waveguide fabrication and characterization Fabrication of the waveguides is performed using electron-beam lithography, reactive ion etching and plasma-enhanced chemical vapour deposition of 2 μm-thick SiO 2 cladding. The fabricated waveguides have a width of 550 nm, height of 300 nm and length of 7 mm, and are characterized by a nonlinear parameter of ∼ 500 W −1 m −1 ( Fig. 1d ). Fibre-to-waveguide coupling losses are 7 dB. The waveguides used for the continuous-wave four-wave-mixing experiments and the optical parametric amplification experiments with the 2.0 ps pulsed-pump utilized waveguides with a loss of ∼ 10 dB cm −1 . Improved waveguides with lower losses of 4.5 dB cm −1 were used in the optical parametric amplification experiments utilizing the 500 fs pulsed pump. Four-wave-mixing and optical parametric amplification experiments The conversion efficiency here is defined as the on/off ratio between the measured signal/idler power at the output of the waveguide with the pump on, and the measured signal power at the output of the waveguide with the pump off [12] , [27] , [43] , [51] , [64] . Optical parametric amplification/gain is achieved when the conversion efficiency exceeds 0 dB. For the continuous-wave four-wave-mixing experiments, a tunable continuous-wave laser is used for the signal. The pump utilizes a tunable continuous-wave laser amplified using a low-noise erbium doped fibre amplifier, followed by a band pass filter to eliminate the amplified spontaneous emission noise outside of the continuous-wave line. The pump and signal are subsequently combined using a wavelength division multiplexer. The output spectra were measured using a grating-based optical spectrum analyser (OSA). The optical parametric amplification experiments utilized a pulsed pump delivering 500 fs or 2.0 ps pulses at a repetition rate of 20 MHz from a fibre laser. Using the measured value of β 2 =0.28 ps 2 m −1 , the dispersion length [21] for 500 fs pulses in the waveguide assuming a sech [2] profile is ∼ 30 cm, around 40 times longer than the physical length of the USRN waveguide, and therefore dispersive effects on the pulse should be negligible. The signal was a tunable continuous-wave laser. The pump and signal were combined using a wavelength division multiplexer and the output spectra were measured using a grating-based OSA. The peak power of the signal peak is calculated as , where R p is the pulse repetition rate of 20 MHz and T pulse is the pulse width [28] , [29] , [42] . P signal, ave ( λ ) represents the average output power spectrum of the signal as a function of wavelength measured by the OSA [37] . In deriving P sig,peak , the power residing in the continuous-wave signal line is subtracted from the spectrum of P signal, ave ( λ ). The peak power in the n th idler is given by , where P idler( n ), ave represents the measured average output power spectrum of the n th idler. The waveguide-output fibre coupling losses are added to obtain the actual signal power out of the waveguide. The on/off optical parametric gain of the signal is calculated as the ratio, P sig, peak / P signal, out , where P signal, out is the CW signal power at the output of the waveguide with the pump off. The on/off optical parametric gain of the n th idler is calculated as the ratio, P idler( n ), peak / P signal, out . Data availability All relevant data are included in the paper and/ or its Supplementary Information files. How to cite this article: Ooi, K. J. A. et al . Pushing the limits of CMOS optical parametric amplifiers with USRN:Si 7 N 3 above the two-photon absorption edge. Nat. Commun. 8, 13878 doi: 10.1038/ncomms13878 (2017). Publisher’s note : Springer Nature remains neutral with regard to jurisdictional claims in published maps and institutional affiliations.